Transcriptional silencing of long noncoding RNAGNG12-AS1uncouples its transcriptional and product-related functions Long noncoding RNAs (lncRNAs) regulate gene expression via their RNA product or through transcriptional interference, yet a strategy to differentiate these two processes is lacking. To address this, we used multiple small interfering RNAs (siRNAs) to silence GNG12-AS1 , a nuclear lncRNA transcribed in an antisense orientation to the tumour-suppressor DIRAS3 . Here we show that while most siRNAs silence GNG12-AS1 post-transcriptionally, siRNA complementary to exon 1 of GNG12-AS1 suppresses its transcription by recruiting Argonaute 2 and inhibiting RNA polymerase II binding. Transcriptional, but not post-transcriptional, silencing of GNG12-AS1 causes concomitant upregulation of DIRAS3 , indicating a function in transcriptional interference. This change in DIRAS3 expression is sufficient to impair cell cycle progression. In addition, the reduction in GNG12-AS1 transcripts alters MET signalling and cell migration, but these are independent of DIRAS3 . Thus, differential siRNA targeting of a lncRNA allows dissection of the functions related to the process and products of its transcription. The mammalian genome encodes many long noncoding RNAs (lncRNAs) that play pivotal roles in gene regulation during development and disease pathogenesis [1] , [2] , [3] . LncRNAs can regulate gene expression through transcriptional interference (TI) [4] , [5] or through the RNA product itself [1] , [2] . TI occurs when the act of transcribing a gene directly interferes with the transcription of an adjacent gene in cis , either at its initiation site or at an essential cis -regulatory element [6] , [7] . Transcription of lncRNA has been shown to interfere with the transcription of adjacent genes by altering the binding of transcription factors [8] , [9] , [10] and/or RNA polymerase II (Pol II) [11] , nucleosome remodelling [12] or inducing changes in histone modifications [13] , [14] . So far, the strategies for demonstrating TI in mammalian cells have relied upon genetic engineering methodologies that remove the promoter region or insert premature transcriptional termination sites within the transcriptional unit [4] . An alternative approach would be to leave the DNA template intact and directly target the lncRNA with small interfering RNAs (siRNAs). It is widely perceived that RNA interference (RNAi) is a cytoplasmic pathway for post-transcriptional gene silencing [15] . However, RNAi-based technology has been used to post-transcriptionally deplete a lncRNA Kcnq1ot1 in the nucleus and demonstrate that this lncRNA product is not required to maintain imprinting of adjacent genes [16] . RNAi has also been shown to induce transcriptional gene silencing (TGS) [17] , [18] , [19] . siRNA-directed TGS can lead to epigenetic changes such as DNA methylation and histone methylation at the target promoters [17] , [20] , [21] , [22] . In addition, promoter-targeting siRNAs can induce TGS by blocking the recruitment and the activity of Pol II (refs 23 , 24 , 25 ). In all these cases, Argonaute proteins (AGO1 and AGO2) were shown to be key players of TGS [21] , [24] , [26] , [27] , [28] , [29] . Finally, it has been shown that siRNAs can be used to knockdown small-nuclear ncRNA 7SK [30] . These observations prompted us to investigate whether siRNAs can be used to inhibit lncRNA transcription and to explore the functional consequences of this process. In particular, we postulated that by targeting different regions of the lncRNA, we could uncouple the act of transcription from the function of the transcript. This would enable us to investigate how lncRNAs regulate adjacent genes in cis through TI. As a model, we used the imprinted tumour-suppressor DIRAS3 locus, where we have recently characterized a novel lncRNA known as GNG12-AS1 (ref. 31 ). GNG12-AS1 is transcribed in an antisense orientation to DIRAS3 and its neighbouring non-imprinted genes GNG12 and WLS ( Fig. 1a ). We have shown that this lncRNA is allele specifically silenced in cancer cell lines depending on the imprinted state of DIRAS3 (ref. 31 ). DIRAS3 (also known as ARHI and NOEY2 ) is a Ras-related imprinted tumour suppressor involved in the inhibition of growth, motility and invasion via several signalling pathways including RAS/MAPK, STAT3 and PI3K [32] . DIRAS3 is downregulated in 70% of breast and ovarian cancer [33] , [34] , [35] , and its loss of expression correlates with cancer progression and metastasis [34] , [35] . The mechanism responsible for DIRAS3 downregulation to date involves different epigenetic mechanisms and loss of heterozygosity [32] . We hypothesized that TI by GNG12-AS1 could represent an additional layer of regulating DIRAS3 dosage. 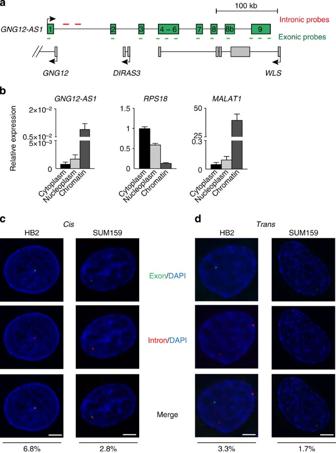Figure 1:GNG12-AS1is a stable lncRNA in the nucleus. (a) Schematic representation of theGNG12-AS1genomic locus (chr1: 68297971–68668670, hg19) relative toGNG12, DIRAS3andWLS. The arrows show the direction of transcription.GNG12-AS1exons are in green and are numbered as previously reported31. Probes used for FISH are marked. Intronic, labelled in red identify the site of transcription. Exonic, labelled in green, mark mature transcripts. (b) RNA distribution from the cytoplasm, nucleoplasm and chromatin in SUM159 cells as quantified by qRT–PCR.RPS18andMALAT1are positive controls for the cytoplasmic and chromatin fraction, respectively. Note enrichment ofGNG12-AS1in the chromatin fraction. Relative RNA levels are standardized to the geometric mean ofGAPDHandβ-actin. Error bars represent the s.e.m. values of three independent experiments. (c,d) Co-localization of exonic (green) and intronic (red)GNG12-AS1probes in HB2 and SUM19 cells by single-molecule RNA FISH.GNG12-AS1associates with its site of transcription (2.8% in SUM159, 6.8% in HB2;cis,c) but is also present at the other sites in the nucleus (1.7% in SUM159, 3.3% in HB2,trans,d). The numbers represent the percentage of cells positive for exonic and intronic FISH signal (n=132 for HB2;n=176 for SUM159). The nucleus was stained with 4,6-diamidino-2-phenylindole (DAPI). Scale bar, 7 μm. Figure 1: GNG12-AS1 is a stable lncRNA in the nucleus. ( a ) Schematic representation of the GNG12-AS1 genomic locus (chr1: 68297971–68668670, hg19) relative to GNG12, DIRAS3 and WLS . The arrows show the direction of transcription. GNG12-AS1 exons are in green and are numbered as previously reported [31] . Probes used for FISH are marked. Intronic, labelled in red identify the site of transcription. Exonic, labelled in green, mark mature transcripts. ( b ) RNA distribution from the cytoplasm, nucleoplasm and chromatin in SUM159 cells as quantified by qRT–PCR. RPS18 and MALAT1 are positive controls for the cytoplasmic and chromatin fraction, respectively. Note enrichment of GNG12-AS1 in the chromatin fraction. Relative RNA levels are standardized to the geometric mean of GAPDH and β-actin . Error bars represent the s.e.m. values of three independent experiments. ( c , d ) Co-localization of exonic (green) and intronic (red) GNG12-AS1 probes in HB2 and SUM19 cells by single-molecule RNA FISH. GNG12-AS1 associates with its site of transcription (2.8% in SUM159, 6.8% in HB2; cis , c ) but is also present at the other sites in the nucleus (1.7% in SUM159, 3.3% in HB2, trans , d ). The numbers represent the percentage of cells positive for exonic and intronic FISH signal ( n =132 for HB2; n =176 for SUM159). The nucleus was stained with 4,6-diamidino-2-phenylindole (DAPI). Scale bar, 7 μm. Full size image Here, we demonstrate that GNG12-AS1 can be transcriptionally silenced with siRNAs complementary to a region proximal to its transcriptional start site (TSS). The transcriptional silencing of GNG12-AS1 , which is mediated by AGO2, leads to upregulation of DIRAS3 transcription in cis , indicating a function in TI. In contrast, targeting GNG12-AS1 at the 3′ end did not affect its nascent transcription, but reduced the lncRNA through post-transcriptional gene silencing and, importantly, did not affect DIRAS3 transcription. We further show different phenotypic effects in cell cycle and migration depending on whether we target the 5′ or 3′ end of GNG12-AS1. Altogether, our results demonstrate that strategic targeting of siRNA to different regions of an lncRNA can enable the discrimination between functions related to its active transcription and that of the RNA product. GNG12-AS1 is a stable lncRNA localized in the nucleus In this study, we used three non-cancer cell lines (HB2, HS27, MCF10A), which we have previously shown to have normal imprinted DIRAS3 expression, and breast cancer cell lines (SUM159, MCF7), where loss of DIRAS3 imprinting leads to biallelic expression (SUM159) or biallelic silencing of DIRAS3 (MCF7). The non-cancer cell lines expressed GNG12-AS1 from both alleles, whereas the cancer cell lines expressed GNG12-AS1 from one allele [31] . We confirmed the relative expression of DIRAS3 , GNG12 , GNG12-AS1 and WLS in these cell lines ( Supplementary Fig. 1a ). Actinomycin D chase experiments indicate that GNG12-AS1 is a stable lncRNA with a half-life between 20 and 25 h ( Supplementary Fig. 1b ). DIRAS3 expression remained unchanged in HB2 and increased in HS27 when cells were treated with Actinomycin D, suggesting an inverse relationship between DIRAS3 and GNG12-AS1 transcription. Despite being a stable lncRNA, GNG12-AS1 has a low transcript volume (20–80 molecules per 100 cells; Supplementary Fig. 1c ). Expression analysis following cell fractionation indicated that GNG12-AS1 is localized within the chromatin ( Fig. 1b ), similar to MALAT1 , a lncRNA known to be associated with chromatin [36] . Using single-molecule RNA fluorescence in situ hybridization (RNA FISH; as described in ref. 37 ), we confirmed that GNG12-AS1 is nuclear in HB2 and SUM159 cells. Exonic probes complementary to all exons showed that GNG12-AS1 transcripts accumulate in the nucleus in discrete foci in 19% of SUM159 and 25% of HB2 cells ( Supplementary Fig. 1d ). Intronic RNA FISH probes complementary to the first intron of GNG12-AS1 were found to co-localize with the exonic signals in about two-thirds of cases where both probes were present in the same cell (6.8% in HB2 cells; 2.8% in SUM159 cells; Fig. 1c ). As intronic probes are usually indicative of nascent transcription and exonic probes can detect both primary and mature transcripts, their co-localization may indicate that the processed transcript remains at its site of transcription, which would fit with GNG12-AS1 being co-transcriptionally spliced, as previously reported [31] . However, as we also see separate signals for exonic and intronic probes, it is likely that some GNG12-AS1 also accumulate at other sites in the nucleus away from its site of transcription (3.3% in HB2 cells; 1.7% in SUM159 cells; Fig. 1d ). A caveat to the interpretation of FISH data is that intronic and exonic RNA FISH probes might not hybridize to nascent and mature lncRNA transcripts in a mutually exclusive way. Nascent RNA contains exons and the mature lncRNAs may be present as unspliced isoforms. In SUM159 cells, the intronic probe mostly produced a single FISH signal (13% of cells being monoallelic, Supplementary Fig. 1e ), which fits with previous pyrosequencing data reporting allele-specific GNG12-AS1 expression in cancer cells [31] . By contrast, in HB2 cells, even though pyrosequencing showed an allelic ratio of 50% (ref. 31 ), we observed cells with both single and double intronic signals (8 and 6% of cells, respectively; Supplementary Fig. 1e ), suggesting that GNG12-AS1 is heterogeneously biallelic and randomly monoallelic at the cellular level in HB2 cells. Together, these data confirm that GNG12-AS1 is a stable lncRNA that is present in the nucleus at distinct foci. TI between GNG12-AS1 and DIRAS3 To investigate the role of GNG12-AS1 , we depleted GNG12-AS1 using siRNAs ( Fig. 2a ). GNG12-AS1 has multiple isoforms [31] , thus we designed siRNAs against several different exons and found that siRNA targeted to exons 1, 5 and 7 reduced GNG12-AS1 by 50–70% in HB2 and SUM159 cells ( Supplementary Fig. 2a–c ). These exons are common to all of the known splice forms of GNG12-AS1 . Using several primer sets to capture the various GNG12-AS1 isoforms, we confirmed that siRNAs against exons 1 and 7 efficiently knockdown GNG12-AS1 ( Supplementary Fig. 2d ). We further confirmed that the knockdown occurred in all cellular compartments ( Supplementary Fig. 2e ). Thus, we are able to deplete GNG12-AS1 in the nucleus with siRNA. 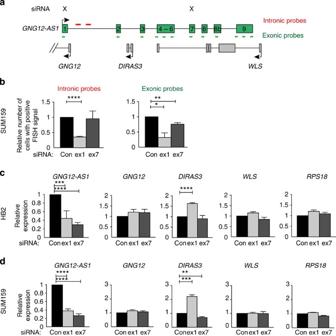Figure 2: Transcriptional interference byGNG12-AS1regulatesDIRAS3. (a) TheGNG12-AS1locus where X indicates the exons targeted by siRNA. (b) Changes in single-molecule RNA FISH signals after treating SUM159 cells with siRNA directed to exon 1 or exon 7 ofGNG12-AS1. Changes in nascent transcription after exon 1, but not exon 7 siRNA, ofGNG12-AS1were found using intronic probes (left panel). Both siRNAs decreased the number of exonic FISH signal (right panel). Cells positive for intronic probes include cells with both mono and biallelic signal, and cells positive for exonic probes include cells having one or more dots. The number of cells positive for RNA FISH signal is presented relative to control siRNA (control siRNA=454 cells; exon 1 siRNA=429 cells; exon 7 siRNA=257 cells). (c,d) siRNA-mediated knockdown of exon 1 (5′ targeting) and exon 7 ofGNG12-AS1(3′ targeting) in HB2 (mammary epithelial cell line,c) and SUM159 (breast cancer cell line,d). Similar results were obtained in two additional cell lines (Supplementary Fig. 3a,b).DIRAS3is upregulated only when the 5' end ofGNG12-AS1is targeted by siRNA directed to exon 1. For all the graphs, expression levels ofDIRAS3, GNG12, WLS, GNG12-AS1were measured by qRT–PCR, normalized toGAPDHor to geometric mean ofGAPDHandRPS18(see alsoSupplementary Fig. 3c–f), and are presented relative to control siRNA. Primers spanning exons 7–8 were used forGNG12-AS1expression.RPS18was used as a negative control gene whose expression does not change upon siRNA treatment. Error bars, s.e.m. (n=3 biological replicates). *P<0.05, **P<0.01, ***P<0.001 and ****P<0.0001 by two-tailed Student’st-test. Figure 2: Transcriptional interference by GNG12-AS1 regulates DIRAS3 . ( a ) The GNG12-AS1 locus where X indicates the exons targeted by siRNA. ( b ) Changes in single-molecule RNA FISH signals after treating SUM159 cells with siRNA directed to exon 1 or exon 7 of GNG12-AS1 . Changes in nascent transcription after exon 1, but not exon 7 siRNA, of GNG12-AS1 were found using intronic probes (left panel). Both siRNAs decreased the number of exonic FISH signal (right panel). Cells positive for intronic probes include cells with both mono and biallelic signal, and cells positive for exonic probes include cells having one or more dots. The number of cells positive for RNA FISH signal is presented relative to control siRNA (control siRNA=454 cells; exon 1 siRNA=429 cells; exon 7 siRNA=257 cells). ( c , d ) siRNA-mediated knockdown of exon 1 (5′ targeting) and exon 7 of GNG12-AS1 (3′ targeting) in HB2 (mammary epithelial cell line, c ) and SUM159 (breast cancer cell line, d ). Similar results were obtained in two additional cell lines ( Supplementary Fig. 3a,b ). DIRAS3 is upregulated only when the 5' end of GNG12-AS1 is targeted by siRNA directed to exon 1. For all the graphs, expression levels of DIRAS3, GNG12, WLS, GNG12-AS1 were measured by qRT–PCR, normalized to GAPDH or to geometric mean of GAPDH and RPS18 (see also Supplementary Fig. 3c–f ), and are presented relative to control siRNA. Primers spanning exons 7–8 were used for GNG12-AS1 expression. RPS18 was used as a negative control gene whose expression does not change upon siRNA treatment. Error bars, s.e.m. ( n =3 biological replicates). * P <0.05, ** P <0.01, *** P <0.001 and **** P <0.0001 by two-tailed Student’s t -test. Full size image RNA FISH analysis in SUM159 cells showed that although siRNAs to either exon 1 or exon 7 effectively ablated GNG12-AS1 detectable with exonic probes, siRNA targeting exon 1 reduced GNG12-AS1 detectable with intronic probes (nascent transcripts) more efficiently than siRNA to exon 7 ( Fig. 2b ). These results indicate that although both siRNAs can efficiently reduce GNG12-AS1 levels in different cellular compartments, siRNA complementary to the 5′ end of GNG12-AS1 may preferentially inhibit its nascent transcription. We next asked whether depletion of GNG12-AS1 affects the transcription of its neighbouring genes. We analysed the expression of GNG12 , DIRAS3 and WLS after depleting GNG12-AS1 with siRNAs against exon 1 and exon 7. DIRAS3, but not GNG12 or WLS, was upregulated after targeting exon 1 of GNG12-AS1 in four cell lines ( Fig. 2c,d and Supplementary Fig. 3a–f ). DIRAS3 upregulation was consistent in different cell lines when GAPDH ( Fig. 2c,d and Supplementary Fig. 3a,b ) or the geometric mean of GAPDH and RPS18 were used ( Supplementary Fig. 3c–f ). Thus, for further quantitative real-time PCR (qRT–PCR) experiments, we used GAPDH as the reference gene. In a fifth cell line MCF7, despite a 60% reduction in GNG12-AS1, expression of DIRAS3 could not be reactivated ( Supplementary Fig. 4a ). In MCF7 cells, DIRAS3 is more hypermethylated at its promoter compared with SUM159 cells [31] . Off-target effects were excluded by the use of additional siRNAs against exon 1 and exon 7 of GNG12-AS1 ( Supplementary Fig. 4b ). Furthermore, we used the randomized nucleotide sequence (scrambled siRNAs) of exon 1 and exon 7 siRNAs ( Supplementary Fig. 4c,d ), as well as C911 mismatch siRNA controls [38] , all of which failed to affect GNG12-AS1 and DIRAS3 levels ( Supplementary Fig. 4e ). To exclude the possibility of GNG12-AS1 regulating DIRAS3 expression in trans , we ectopically introduced GNG12-AS1 in SUM159 and HB2 cells. Overexpression of the most common splice variants of GNG12-AS1 had no effect on expression of DIRAS3 or the surrounding genes ( Supplementary Fig. 5a,b ). As DIRAS3 is an imprinted gene, we examined whether allele-specific expression changed after GNG12-AS1 depletion. DIRAS3 imprinting and its methylation status were unaltered ( Supplementary Fig. 5c–e ). Taken together, these results suggest that GNG12-AS1 modulates the expression of the already active DIRAS3 allele in cis and that siRNA to exon 1 of GNG12-AS1 disrupts this function without affecting expression of neighbouring genes. siRNA against 5′ end of GNG12-AS1 blocks RNA Pol II Next, we examined whether inhibition of DIRAS3 in cis can be achieved by targeting GNG12-AS1 exons closer to the DIRAS3 gene. Similar to when we targeted exon 7, siRNA to exon 5 efficiently reduced GNG12-AS1 ( Supplementary Fig. 2b,c ), but did not upregulate DIRAS3 ( Supplementary Fig. 6a,b ). In one of the cell lines, siRNA to exon 5 led to WLS downregulation. siRNAs to exons 2 and 3, which flank DIRAS3 on either side, reduced GNG12-AS1 isoform specifically ( Supplementary Fig. 2f,g ), suggesting that these siRNAs function post-transcriptionally. These siRNAs had no effect on DIRAS3 expression further supporting modulation via the act of transcription rather than through a specific GNG12-AS1 isoform ( Supplementary Fig. 6c,d ). To prove that the cis function of GNG12-AS1 is modulated by siRNA targeting exon 1, which leads to the inhibition of TI between GNG12-AS1 and DIRAS3 , we profiled Pol II and histone modifications. As shown in Fig. 3a,b , a significant reduction in Pol II binding was observed at the TSS of GNG12-AS1 when exon 1, but not exon 7, was targeted by siRNA. Concomitantly, an increase in Pol II binding was observed at the DIRAS3 TSS. Nuclear run-on assays showed that the reduction in Pol II binding was associated with reduced nascent GNG12-AS1 transcription. Thus, a reduction of GNG12-AS1 and increased DIRAS3 run-on transcripts were observed with siRNA targeting exon 1, but not exon 7 ( Fig. 3c ). 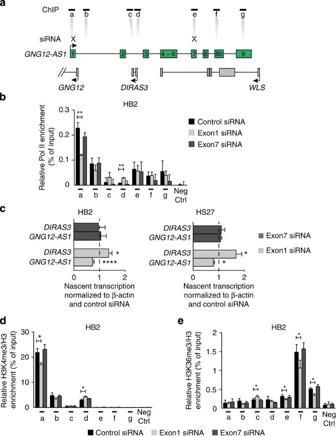Figure 3: Inhibition of Pol II after siRNA targeted to exon 1 ofGNG12-AS1. (a) TheGNG12-AS1locus showing the location of primer sets (a–g) used for chromatin immunoprecipitation (ChIP) analysis.GNG12-AS1TSS (a), region 1.6 kb downstream ofGNG12-AS1TSS (b), exon 2 ofDIRAS3(c),DIRAS3TSS (d),GNG12-AS1exon 7 (e),GNG12-AS1exon 8b (f) andGNG12-AS1exon 9 (g). The X indicates the exons where siRNAs were targeted. (b) Pol II ChIP analysis in HB2 cells treated with siRNA to exons 1 or 7 and controls. ChIP enrichments are presented as the percentage of protein bound, normalized to input. siRNA targeting exon 1 ofGNG12-AS1, but not exon 7, results in reduced Pol II binding atGNG12-AS1TSS (a). At the same time, increased Pol II binding was observed at theDIRAS3TSS (d). (c) Nuclear run-on analysis ofGNG12-AS1andDIRAS3transcription after treatment of HB2 cells (left panel) or HS27 cells (right panel) with control and exon 1 or exon 7GNG12-AS1siRNA. siRNA targeting exon 1 results in reducedGNG12-AS1nascent transcription, which leads to increasedDIRAS3transcription. Data are normalized toβ-actinand standardized to control siRNA, which is set up as 1 and shown as dotted line. (d,e) ChIP analysis from HB2 cells treated with siRNA to exons 1 or 7 using H3K4me3 (d) and H3K36me3 (e) antibodies. The precipitated DNA fragments were subjected to qRT–PCR analysis with the same primers as for Pol II ChIP. siRNA targeting exon 1, but not exon 7, ofGNG12-AS1reduced H3K4me3 atGNG12-AS1TSS (a) and H3K36me3 levels in the body ofGNG12-AS1(e–g). Concomitantly, H3K4me3 and H3K36me3 levels increased at theDIRAS3(d,c, respectively). Levels of H3K4me3 and H3K36me3 were normalized to histone H3 density. For all the graphs, ChIP enrichments are presented as the percentage of protein bound, normalized to input. Neg ctrl=negative control region. Error bars, s.e.m. (n=3 biological replicates). *P<0.05, **P<0.01 and ****P<0.0001 by two-tailed Student’st-test. Figure 3: Inhibition of Pol II after siRNA targeted to exon 1 of GNG12-AS1 . ( a ) The GNG12-AS1 locus showing the location of primer sets (a–g) used for chromatin immunoprecipitation (ChIP) analysis. GNG12-AS1 TSS (a), region 1.6 kb downstream of GNG12-AS1 TSS (b), exon 2 of DIRAS3 (c), DIRAS3 TSS (d), GNG12-AS1 exon 7 (e), GNG12-AS1 exon 8b (f) and GNG12-AS1 exon 9 (g). The X indicates the exons where siRNAs were targeted. ( b ) Pol II ChIP analysis in HB2 cells treated with siRNA to exons 1 or 7 and controls. ChIP enrichments are presented as the percentage of protein bound, normalized to input. siRNA targeting exon 1 of GNG12-AS1 , but not exon 7, results in reduced Pol II binding at GNG12-AS1 TSS (a). At the same time, increased Pol II binding was observed at the DIRAS3 TSS (d). ( c ) Nuclear run-on analysis of GNG12-AS1 and DIRAS3 transcription after treatment of HB2 cells (left panel) or HS27 cells (right panel) with control and exon 1 or exon 7 GNG12-AS1 siRNA. siRNA targeting exon 1 results in reduced GNG12-AS1 nascent transcription, which leads to increased DIRAS3 transcription. Data are normalized to β-actin and standardized to control siRNA, which is set up as 1 and shown as dotted line. ( d , e ) ChIP analysis from HB2 cells treated with siRNA to exons 1 or 7 using H3K4me3 ( d ) and H3K36me3 ( e ) antibodies. The precipitated DNA fragments were subjected to qRT–PCR analysis with the same primers as for Pol II ChIP. siRNA targeting exon 1, but not exon 7, of GNG12-AS1 reduced H3K4me3 at GNG12-AS1 TSS (a) and H3K36me3 levels in the body of GNG12-AS1 (e–g). Concomitantly, H3K4me3 and H3K36me3 levels increased at the DIRAS3 (d,c, respectively). Levels of H3K4me3 and H3K36me3 were normalized to histone H3 density. For all the graphs, ChIP enrichments are presented as the percentage of protein bound, normalized to input. Neg ctrl=negative control region. Error bars, s.e.m. ( n =3 biological replicates). * P <0.05, ** P <0.01 and **** P <0.0001 by two-tailed Student’s t -test. Full size image To determine whether we could ablate unspliced transcripts and if so, whether this could affect DIRAS3 expression, we designed siRNAs to the first intron at 195 and 2,933 bp downstream of the GNG12-AS1 TSS. In both HB2 and HS27 cell lines, these siRNAs resulted in a reduction of GNG12-AS1 , indicating that the unspliced GNG12-AS1 transcript can be targeted by siRNA. However, increased DIRAS3 expression occurred only in HS27 cells ( Supplementary Fig. 7a,d ), indicating that siRNA specifically targeting exon 1 is more efficient at disrupting the regulatory relationship between GNG12-AS1 and DIRAS3 transcription. Consistent with the changes in Pol II binding, we observed changes in active histone modifications when GNG12-AS1 was depleted using siRNA against exon 1, but not with exon 7 ( Fig. 3d,e ). Histone H3 lysine 4 trimethylation (H3K4me3) was reduced at the GNG12-AS1 TSS and increased at the DIRAS3 TSS. Furthermore, histone H3 lysine 36 trimethylation (H3K36me3), a marker for Pol II elongation [39] , was decreased in the body of GNG12-AS1 and increased within DIRAS3 . As GNG12-AS1 depletion with exon 1 siRNA did not affect WLS expression, a reduction in H3K36me3 at 3′ end of GNG12-AS1 correlates with reduction in its transcriptional activity. The reduction of active histone modifications at the GNG12-AS1 TSS was not accompanied by a reciprocal increase of silencing modifications previously reported to be involved in TGS [20] , [21] , [29] , such as histone H3 lysine 9 trimethylation (H3K9me3) and histone H3 lysine 27 trimethylation (H3K27me3; Supplementary Fig. 8a,b ). In addition, DNA methylation was unchanged at the GNG12-AS1 TSS ( Supplementary Fig. 8c ). The changes in Pol II binding at the TSS of GNG12-AS1 , together with the changes in active histone modifications associated with transcriptional activity after siRNA to exon 1, suggest that targeting the 5′ end of this lncRNA results in transcriptional silencing. However, to date, in all instances of TGS with exogenous siRNAs in human cells, the siRNAs were directed to the gene promoters. We therefore designed two siRNAs targeting GNG12-AS1 upstream of the TSS (33 and 129 bp upstream of TSS). These siRNAs had no effect on GNG12-AS1 expression ( Supplementary Fig. 7c,d ), suggesting that transcription needs to be initiated for effective knockdown of the lncRNA. In summary, siRNA targeting specifically exon 1 of GNG12-AS1 reduced its nascent transcription, without inducing changes in silent chromatin marks. Nevertheless, reduced transcription was associated with diminished Pol II activity and the redistribution of active histone marks, which led to increased DIRAS3 expression. AGO2 mediates transcriptional inhibition of GNG12-AS1 As TGS is achieved through the RNAi machinery [24] , [25] , [27] , [28] , we investigated whether siRNA-mediated silencing of GNG12-AS1 involves Argonaute proteins. First, we examined whether the reduction in GNG12-AS1 transcript by siRNA targeted to exon 1 could be rescued by depletion of AGO1/2 proteins. We found that depletion of AGO2 rescued GNG12-AS1 expression in cells exposed to siRNAs against exon 1 and exon 7 and abolished DIRAS3 upregulation in cells treated with siRNA against exon 1 ( Fig. 4a ). This effect was specific to AGO2, as AGO1 depletion did not rescue GNG12-AS1 depletion or DIRAS3 levels ( Supplementary Fig. 9a ). Similar results were obtained in the HS27 cell line ( Supplementary Fig. 9b,c ), confirming that AGO2 is involved in both the transcription- and post-transcription-mediated mechanism of siRNA-directed downregulation of GNG12-AS1. 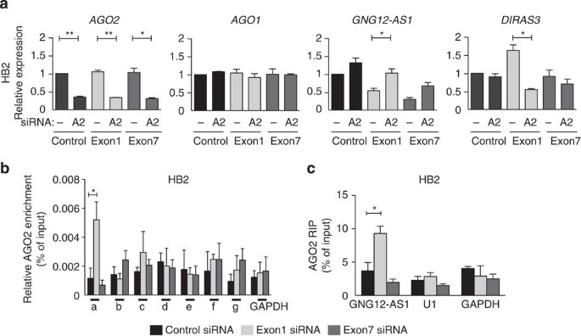Figure 4:AGO2mediates transcriptional inhibition ofGNG12-AS1. (a) HB2 cells were transfected with siRNA to exon 1 or exon 7 ofGNG12-AS1together with control siRNA and siRNA targetingAGO2(A2) (a) orAGO1(A1) (Supplementary Fig. 9a). Expression levels ofAGO2, AGO1, DIRAS3andGNG12-AS1were normalized toGAPDHand compared with control siRNA by qRT–PCR.AGO1levels were not affected by either singleAGO2siRNA or double knockdown ofAGO2andGNG12-AS1. Transcriptional upregulation ofDIRAS3can be rescued by depletion ofAGO2and siRNA targeting exon 1 ofGNG12-AS1,whereas siRNA-mediated reduction ofGNG12-AS1with both siRNAs expression can be rescued by depletion of AGO2. (b) AGO2 ChIP analysis in HB2 cells after siRNA depletion ofGNG12-AS1. Thexaxis shows enrichment of AGO2 at regions described inFig. 3a. AGO2 binding was enriched only at the TSS ofGNG12-AS1(a) after siRNA to exon 1. TheGAPDHTSS was used as negative control region for AGO2 ChIP. (c) RIP from nuclear HB2 extracts showing association of AGO2 withGNG12-AS1transcript after treatment of cells with exon 1 but not exon 7 siRNA.U1andGAPDHwere used as negative control RNAs for AGO2 RIP. RIP enrichments are presented as % of input RNA. For all the graphs, error bars indicate s.e.m. (n=3 biological replicates). *P<0.05 and **P<0.01 by two-tailed Student’st-test. Figure 4: AGO2 mediates transcriptional inhibition of GNG12-AS1 . ( a ) HB2 cells were transfected with siRNA to exon 1 or exon 7 of GNG12-AS1 together with control siRNA and siRNA targeting AGO2 (A2) ( a ) or AGO1 (A1) ( Supplementary Fig. 9a ). Expression levels of AGO2, AGO1, DIRAS3 and GNG12-AS1 were normalized to GAPDH and compared with control siRNA by qRT–PCR. AGO1 levels were not affected by either single AGO2 siRNA or double knockdown of AGO2 and GNG12-AS1 . Transcriptional upregulation of DIRAS3 can be rescued by depletion of AGO2 and siRNA targeting exon 1 of GNG12-AS1, whereas siRNA-mediated reduction of GNG12-AS1 with both siRNAs expression can be rescued by depletion of AGO2. ( b ) AGO2 ChIP analysis in HB2 cells after siRNA depletion of GNG12-AS1 . The x axis shows enrichment of AGO2 at regions described in Fig. 3a . AGO2 binding was enriched only at the TSS of GNG12-AS1 ( a ) after siRNA to exon 1. The GAPDH TSS was used as negative control region for AGO2 ChIP. ( c ) RIP from nuclear HB2 extracts showing association of AGO2 with GNG12-AS1 transcript after treatment of cells with exon 1 but not exon 7 siRNA. U1 and GAPDH were used as negative control RNAs for AGO2 RIP. RIP enrichments are presented as % of input RNA. For all the graphs, error bars indicate s.e.m. ( n =3 biological replicates). * P <0.05 and ** P <0.01 by two-tailed Student’s t -test. Full size image We verified that AGO2 is present in the nucleus and cytoplasm ( Supplementary Fig. 9d ), as previously reported [18] . Next, we used chromatin immunoprecipitation (ChIP) analysis to see whether AGO2 associates with the GNG12-AS1 locus. We found that AGO2 was recruited to the GNG12-AS1 TSS only after treatment with siRNA directed to exon 1, but not exon 7 ( Fig. 4b ). This result suggests that AGO2 facilitates the physical interaction between exogenous siRNA to exon 1 and the chromatin to potentially mediate TGS of GNG12-AS1 . Finally, we tested whether GNG12-AS1 associates with AGO2 in the nucleus. RNA immunoprecipitation (RIP) for AGO2 in nuclear extracts transfected with siRNAs showed an interaction between GNG12-AS1 and AGO2 only when siRNA targeted exon 1, and not exon 7 ( Fig. 4c ). Taken together, these results demonstrate that AGO2 mediates transcriptional silencing of GNG12-AS1 by siRNA complementary to exon 1. Cell cycle regulation by GNG12-AS1 DIRAS3 has been implicated in cell cycle regulation [40] , so we next asked if expression levels of DIRAS3 and GNG12-AS1 might correlate at different stages of the cell cycle. We synchronized cells with a double thymidine block ( Fig. 5a ), which arrest cells in S-phase and used cyclin E1 (G1/S transition marker) to monitor cell cycle progression ( Fig. 5c ). An increase in GNG12-AS1 transcription was observed after the release from double thymidine block, which coincided with the downregulation of DIRAS3. Cell cycle synchronization using serum starvation, followed by release with serum-containing media, showed similar results ( Fig. 5b,d ). The inverse relationship between expression levels of GNG12-AS1 and DIRAS3 , which was tightly maintained throughout the cell cycle, further supports the evidence that GNG12-AS1 transcription modulates DIRAS3 expression in cis through TI. 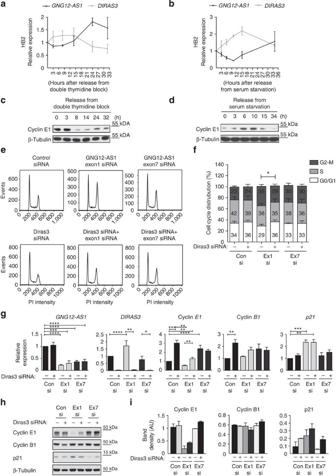Figure 5:DIRAS3-dependent and independent cell cycle regulation. (a,b) Expression patterns ofGNG12-AS1andDIRAS3are inversely correlated in synchronized cells. HB2 cells were synchronized by double thymidine block (a) or serum starvation (b) and released at indicated time points. Expression levels were measured by qRT–PCR, normalized toGAPDHand standardized to time point 0 h (set as 1). Error bars, s.e.m. (n=3 biological replicates). (c,d) Immunoblot of cyclin E1 (G1/S transition marker) was used to monitor cell cycle progression of HB2 cells synchronized with a double thymidine block (c) or serum starvation (d). β-Tubulin was used as a loading control. (e) FACS analysis of asynchronous HB2 cells after depletion ofGNG12-AS1,DIRAS3or simultaneous depletion ofGNG12-AS1andDIRAS3. The histograms are representative images of four biological replicates. (f) Cell cycle distribution of HB2 cells following siRNA conditions as shown ine. Note the restoration of G1 cell number betweenGNG12-AS1exon 1 siRNA-treated cells and simultaneous depletion ofGNG12-AS1andDIRAS3(control siRNA: 34% versus exon 1 siRNA: 29%, *P<0.05 by two-tailed Student’st-test). Increase in G2/M population was observed between control and exon 1 siRNA (control siRNA: 23% versus exon 1 siRNA: 35%, ***P<0.001) and exon 7 siRNA (control siRNA: 23% versus exon 7 siRNA: 30%, *P<0.05 by two-tailed Student’st-test). (g) qRT–PCR ofDIRAS3, GNG12-AS1, cyclin E1, cyclin B1andp21afterGNG12-AS1andDIRAS3depletion as shown ine. Expression levels are normalized toGAPDHand presented relative to control siRNA. Error bars, s.e.m. (n=4 biological replicates). *P<0.05, **P<0.01, ***P<0.001 and ****P<0.0001 by two-tailed Student’st-test. (h) Immunoblot of cyclin E1, cyclin B1 and p21 afterGNG12-AS1andDIRAS3depletion in HB2 cells. Cyclin E1 was reduced only in exon 1 siRNA-treated cells and partially rescued after simultaneous depletion ofGNG12-AS1andDIRAS3(compare lane 3 to lane 4). β-Tubulin was used as a loading control. (i) Quantification of immunoblots from (h;n=2 biological replicates). Figure 5: DIRAS3 -dependent and independent cell cycle regulation. ( a , b ) Expression patterns of GNG12-AS1 and DIRAS3 are inversely correlated in synchronized cells. HB2 cells were synchronized by double thymidine block ( a ) or serum starvation ( b ) and released at indicated time points. Expression levels were measured by qRT–PCR, normalized to GAPDH and standardized to time point 0 h (set as 1). Error bars, s.e.m. ( n =3 biological replicates). ( c , d ) Immunoblot of cyclin E1 (G1/S transition marker) was used to monitor cell cycle progression of HB2 cells synchronized with a double thymidine block ( c ) or serum starvation ( d ). β-Tubulin was used as a loading control. ( e ) FACS analysis of asynchronous HB2 cells after depletion of GNG12-AS1 , DIRAS3 or simultaneous depletion of GNG12-AS1 and DIRAS3 . The histograms are representative images of four biological replicates. ( f ) Cell cycle distribution of HB2 cells following siRNA conditions as shown in e . Note the restoration of G1 cell number between GNG12-AS1 exon 1 siRNA-treated cells and simultaneous depletion of GNG12-AS1 and DIRAS3 (control siRNA: 34% versus exon 1 siRNA: 29%, * P <0.05 by two-tailed Student’s t -test). Increase in G2/M population was observed between control and exon 1 siRNA (control siRNA: 23% versus exon 1 siRNA: 35%, *** P <0.001) and exon 7 siRNA (control siRNA: 23% versus exon 7 siRNA: 30%, * P <0.05 by two-tailed Student’s t -test). ( g ) qRT–PCR of DIRAS3, GNG12-AS1, cyclin E1, cyclin B1 and p21 after GNG12-AS1 and DIRAS3 depletion as shown in e . Expression levels are normalized to GAPDH and presented relative to control siRNA. Error bars, s.e.m. ( n =4 biological replicates). * P <0.05, ** P <0.01, *** P <0.001 and **** P <0.0001 by two-tailed Student’s t -test. ( h ) Immunoblot of cyclin E1, cyclin B1 and p21 after GNG12-AS1 and DIRAS3 depletion in HB2 cells. Cyclin E1 was reduced only in exon 1 siRNA-treated cells and partially rescued after simultaneous depletion of GNG12-AS1 and DIRAS3 (compare lane 3 to lane 4). β-Tubulin was used as a loading control. ( i ) Quantification of immunoblots from ( h ; n =2 biological replicates). Full size image We next examined the consequence of upregulating DIRAS3 after inhibiting GNG12-AS1. When GNG12-AS1 was depleted with exon 1 siRNA, we observed a small decrease in G1 cell number (control siRNA: 34% versus exon 1 siRNA: 29%; P =0.0575; Fig. 5e,f ). This result was confirmed by qRT–PCR and immunoblot analysis, which showed decreased cyclin E1 levels ( Fig. 5g–i ). As expected, by combining siRNAs to DIRAS3 and exon 1 siRNA, we were able to neutralize the increase in DIRAS3 expression ( Fig. 5g–i ), which led to a modest but significant restoration of the G1 population (exon 1 siRNA: 29% versus exon 1/DIRAS3 siRNA: 36%, P =0.0105; Fig. 5f ). Analysis of cyclin E1 levels showed that the reduction in G1 cell numbers could be partially rescued with the simultaneous depletion of GNG12-AS1 and DIRAS3 ( Fig. 5g–i ). By contrast, cyclin B1 levels did not differ among GNG12-AS1- and DIRAS3 siRNA-treated cells. Both RNA and protein levels of the cell cycle inhibitor p21 increased when the cells were treated with siRNA to exon 1 in a DIRAS3- independent manner. S-phase distribution was unchanged after reducing GNG12-AS1 . However, both exon 1 and exon 7 siRNAs increased the G2/M population (control siRNA: 23% versus exon 1 siRNA: 35%, P =0.0009; or versus exon 7 siRNA: 30%, P =0.0126). As the increase in G2/M population occurred upon simultaneous depletion of GNG12-AS1 and DIRAS3 (control siRNA: 23% versus exon 1/DIRAS3 siRNA: 29%, P =0.0169; or versus exon 7/DIRAS3 siRNA: 30%, P =0.0084), we concluded that this G2/M delay is a DIRAS3 -independent event. Taken together, these data indicate that GNG12-AS1 has a dual function in controlling cell cycle progression. Transcription of GNG12-AS1 influences the G1 phase of the cell cycle by modulating DIRAS3 expression, whereas the effect on G2/M phase of the cell cycle by GNG12-AS1 is a DIRAS3- independent event, and most likely represents the function of the RNA product. GNG12-AS1 has a trans function regulating cell migration DIRAS3 overexpression has been linked to cell migration and cell proliferation [32] , so we assayed these cellular phenotypes after GNG12-AS1 knockdown. We found that reducing GNG12-AS1 with either of the siRNAs increased cell migration ( Fig. 6a ). As no difference was seen between the two siRNAs, we conclude that these phenotypic effects are due to the reduction of GNG12-AS1 transcripts and independent of DIRAS3 . Indeed, a change in the migration phenotype was also observed in MCF7 cells, where DIRAS3 silencing cannot be reversed by GNG12-AS1 depletion ( Fig. 6a ). We next profiled global transcription changes after knockdown of GNG12-AS1 and found that both siRNAs against this lncRNA induced significant changes in cell adhesion and actin cytoskeleton pathways ( Supplementary Fig. 10a,b ). We focused on mesenchymal epithelial transition factor (MET), a tyrosine kinase receptor for the hepatocyte growth factor, known to regulate cell migration and invasion [41] , [42] and found increased levels of MET ( Fig. 6b,c and Supplementary Fig. 10c ). In line with MET activation, we found elevated levels of the MET downstream target MAP2K4 (mitogen-activated protein kinase kinase 4) [42] . This suggests that activation of MET signalling and its downstream targets could be responsible for the observed changes in cell migration. Interestingly, reducing specific minor isoforms of GNG12-AS1 containing exons 2 and 3 was sufficient to trigger activation of this signalling pathway. Future research into the secondary structure of the GNG12-AS1 will determine if this function is isoform specific. Finally, we examined whether simultaneously depleting GNG12-AS1 and DIRAS3 would prevent MET activation. Increased MET protein levels were maintained, confirming that GNG12-AS1 regulates MET signalling independently of DIRAS3 ( Supplementary Fig. 10d ). Altogether, these data indicate that the GNG12-AS1 transcript inhibits cell migration. In this context, GNG12-AS1 may have a tumour-suppressor function in addition to a role in modulating the expression levels of DIRAS3. 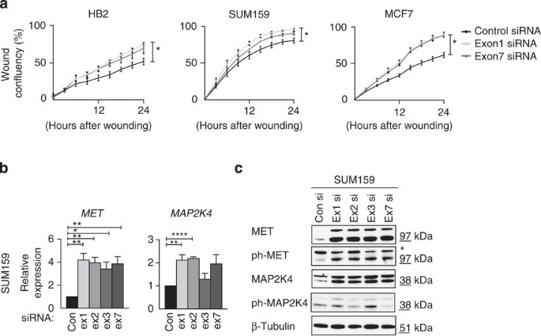Figure 6:GNG12-AS1regulates cell migration independently ofDIRAS3. (a) Cell migration is increased in HB2, SUM159 and MCF7 cells afterGNG12-AS1depletion. Cells were treated with control, exon 1 and exon 7GNG12-AS1siRNAs for 48 h before the wound-healing assay was performed over 24 h time course. Cells depleted with siRNA targeted to exon 1 and exon 7 ofGNG12-AS1have significantly increased cell migration. (b) Validation of gene expression changes in SUM159 cells after depletion ofGNG12-AS1with siRNAs targeting exons 1 and 7. Expression levels ofMETandMAP2K4were measured by qRT–PCR, normalized toGAPDHand compared with control siRNA. The knockdown efficiency ofGNG12-AS1is shown inSupplementary Fig. 2b,f. (c) Immunoblot of MET, MAP2K4 and their active phosphorylated (ph) forms in SUM159 cells after depletion ofGNG12-AS1with siRNAs targeting exons 1, 2, 3 and 7. Asterisk (*) indicates a non-specific band detected with an antibody specific to phosphorylated MET. β-Tubulin was used as a loading control. For all the graphs, error bars indicate s.e.m. (n=3 biological replicates). *P<0.05, **P<0.01 and ****P<0.0001 by two-tailed Student’st-test. Figure 6: GNG12-AS1 regulates cell migration independently of DIRAS3 . ( a ) Cell migration is increased in HB2, SUM159 and MCF7 cells after GNG12-AS1 depletion. Cells were treated with control, exon 1 and exon 7 GNG12-AS1 siRNAs for 48 h before the wound-healing assay was performed over 24 h time course. Cells depleted with siRNA targeted to exon 1 and exon 7 of GNG12-AS1 have significantly increased cell migration. ( b ) Validation of gene expression changes in SUM159 cells after depletion of GNG12-AS1 with siRNAs targeting exons 1 and 7. Expression levels of MET and MAP2K4 were measured by qRT–PCR, normalized to GAPDH and compared with control siRNA. The knockdown efficiency of GNG12-AS1 is shown in Supplementary Fig. 2b,f . ( c ) Immunoblot of MET, MAP2K4 and their active phosphorylated (ph) forms in SUM159 cells after depletion of GNG12-AS1 with siRNAs targeting exons 1, 2, 3 and 7. Asterisk (*) indicates a non-specific band detected with an antibody specific to phosphorylated MET. β-Tubulin was used as a loading control. For all the graphs, error bars indicate s.e.m. ( n =3 biological replicates). * P <0.05, ** P <0.01 and **** P <0.0001 by two-tailed Student’s t -test. Full size image LncRNAs can function via their RNA product and through the act of their transcription. So far it has been challenging to tease apart these two processes. Here we employed an siRNA-based strategy targeting different regions of GNG12-AS1 and found that siRNA selectively targeting the first exon of GNG12-AS1 resulted in increased expression of DIRAS3 in cis . These findings, together with inverse relationship between GNG12-AS1 and DIRAS3 during the cell cycle and Actinomycin D treatment, indicate that the act of transcribing GNG12-AS1 regulates expression of the active DIRAS3 allele by TI. We subsequently showed that this transcriptional targeting by siRNA to the 5′ end of GNG12-AS1 is mediated by AGO2, which binds to the GNG12-AS1 TSS as well as to its transcript. Finally, distinct functional consequences were uncovered, depending on whether GNG12-AS1 transcription was disrupted or whether its product was depleted. The first suggestion that siRNA targeting exon 1 of GNG12-AS1 reduced its nascent transcription was with RNA-FISH, where we observed reduced hybridization with intronic probes after treating cells with this siRNA. More concrete biochemical evidence of transcriptional inhibition were demonstrated by decreased Pol II binding at the GNG12-AS1 TSS with ChIP and reduced nascent transcription with nuclear run-on experiments. siRNA targeted to exon 7, while still reducing the overall GNG12-AS1 product, does not upregulate DIRAS3 and does not change Pol II binding, making this siRNA an excellent internal control for our experiments. Consistent with the data on Pol II binding and nascent transcription, we detected a reduction in the active histone modification, H3K4me3 at the GNG12-AS1 TSS when GNG12-AS1 was depleted using siRNA against exon 1, but not with exon 7. Similarly, the histone modification mark H3K36me3, which normally accumulates in gene body where it is associated with transcriptional elongation [39] , was reduced at the 3′ end of GNG12-AS1 . Thus, our findings suggest that siRNA targeting the 5′ end of GNG12-AS1 led to inhibition of transcriptional initiation and elongation of GNG12-AS1 by directly interfering with Pol II dynamics without inducing changes in DNA methylation and repressive histone marks. To date, all reported cases of exogenous TGS in human cells have used siRNAs against the gene promoter regions or the TSS [17] , [20] , [24] , [25] , [29] . Our study is, therefore, the first to show that targeting the first exon interferes with the transcription of a lncRNA. Indeed, with GNG12-AS1 , targeting regions upstream of the TSS had no effect on its transcription, suggesting that transcription needs to be initiated in order to be targeted by siRNA. This may also explain why, although we found a reduction in active histone modifications, we did not observe an increase in repressive chromatin marks. As TGS is achieved through the RNAi machinery [24] , [25] , [27] , [28] , we investigated the engagement of AGO2 in the inhibition of GNG12-AS1 transcription. siRNAs are known to form a complex with AGO2 in the cytoplasm and then shuffle between the cytoplasm and nucleus [43] . Small-RNA loading is a cytoplasmic process necessary for the nuclear import of AGO2 (refs 18 , 43 , 44 ). It has further been suggested that small RNAs can guide AGO2 to the promoters of ncRNAs and affect their transcription [45] , [46] . Based on these precedents, we would expect that all siRNAs in our experiments would have a similar knockdown efficiency in different cellular compartments, and once the AGO2–siRNA complex was in the nucleus, the functional consequences of the GNG12-AS1 depletion would depend on the region targeted. The presence of AGO2–siRNA complexes in the nucleus and cytoplasm would explain why we could rescue the GNG12-AS1 expression in double knockdown experiments between GNG12-AS1 and AGO2. However, AGO2-siRNA- GNG12-AS1 complexes at the GNG12-AS1 TSS could only be detected in the nucleus when the siRNA was directed to exon 1. As described above, GNG12-AS1 could only be reduced when sequences downstream of its TSS were targeted by siRNA. This finding, together with the RIP results, showing that AGO2 associates with the GNG12-AS1 when cells are treated with siRNA to exon 1, suggest that transcription needs to have been already initiated for siRNA-mediated repression of transcription. Although AGO2–siRNA interactions with chromatin and the lncRNA could be demonstrated by ChIP and RIP, respectively, we do not have direct evidence for siRNA–AGO2 attaching the nascent lncRNA to the chromatin. We propose a model described in Fig. 7 , where exogenous siRNA complementary to the 5′ end (exon 1) of GNG12-AS1 recruits AGO2 to GNG12-AS1 and to the chromatin at its TSS. This complex, containing the siRNA and GNG12-AS1 and possibly other proteins, stalls transcription of GNG12-AS1 by Pol II. DIRAS3 expression is enhanced as a consequence of reduced GNG12-AS1 transcription. 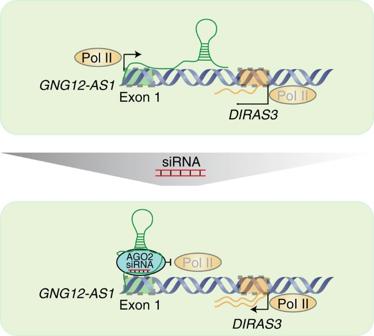Figure 7: Inhibition of transcriptional interference with siRNA. The top panel depicts howGNG12-AS1modulates the expression of the activeDIRAS3allele through transcriptional interference.GNG12-AS1may act as a rheostat forDIRAS3transcription rate. The lower panel depicts how exogenous siRNA molecules in a complex with AGO2 can bind to both the TSS andGNG12-AS1to inhibit Pol II, and block further transcription initiation and elongation ofGNG12-AS1. As a result of transcriptional silencingof GNG12-AS1,transcriptional interference is reduced leading to increased transcription ofDIRAS3. Figure 7: Inhibition of transcriptional interference with siRNA. The top panel depicts how GNG12-AS1 modulates the expression of the active DIRAS3 allele through transcriptional interference. GNG12-AS1 may act as a rheostat for DIRAS3 transcription rate. The lower panel depicts how exogenous siRNA molecules in a complex with AGO2 can bind to both the TSS and GNG12-AS1 to inhibit Pol II, and block further transcription initiation and elongation of GNG12-AS1 . As a result of transcriptional silencing of GNG12-AS1, transcriptional interference is reduced leading to increased transcription of DIRAS3 . Full size image There are two possible mechanisms whereby an exogenous siRNA in a complex with AGO2 could lead to decreased GNG12-AS1 transcription. AGO2 has slicer activity [47] and this could promote cleavage and degradation of the nascent GNG12-AS1. Alternatively, the AGO2–siRNA complex could present a physical block for Pol II initiation and elongation at the GNG12-AS1 TSS. Indeed, AGO2 has been shown to guide small RNAs to inhibit Pol II recruitment and elongation in human cells [24] , [48] independently of its slicer activity [24] , [27] , [45] , [46] . AGO2 has been reported to form a complex with different chromatin-modifying proteins to mediate gene silencing [49] . It is therefore possible that AGO2–siRNA– GNG12-AS1 complexes at the TSS may include further proteins that influence Pol II kinetics. Our model does not distinguish between these different but not necessarily mutually exclusive mechanisms. Silencing of imprinted genes is frequently achieved by TI of an antisense lncRNA [11] , [50] . In these cases, the lncRNA is reciprocally imprinted relative to its target gene and is expressed on the opposite allele. Unlike, the other imprinted genes, we found that it was the already actively expressing DIRAS3 allele being upregulated after GNG12-AS1 knockdown, indicating that GNG12-AS1 has a role in modulating DIRAS3 expression in cis , rather than maintaining its imprinting. A reduction of Pol II and H3K4me3 at the TSS of GNG12-AS1 was associated with a concomitant increase at the DIRAS3 TSS. These shifts reflect the change in dynamics between these two genes as transcription inhibition by the GNG12-AS1 is eased and DIRAS3 transcription is augmented. TI between GNG12-AS1 and DIRAS3 could only be consistently inhibited when siRNAs were target within the first exon of GNG12-AS1 . Targeting the adjacent intron did not lead to DIRAS3 upregulation in both of the cell lines tested. As GNG12-AS1 was efficiently reduced, we presume the nascent transcript was targeted, but GNG12-AS1 may also be present as mature unspliced transcripts that can be targeted post-transcriptionally. There are several enhancer signature peaks (histone H3 lysine 4 monomethylation (H3K4me1) and histone H3 lysine 27 acetylation (H3K27ac)) within this intron as annotated in the ENCODE database ( Supplementary Fig. 11 ). It is possible that although the nascent RNA can be inhibited by siRNA targeted to this region, enough transcription has already occurred through the region to prevent DIRAS3 upregulation. In a region with multiple enhancers, some are likely to be tissue specific, which could explain why DIRAS3 expression is differentially upregulated in two different cell lines. The presence of enhancer marks at this locus would fit with GNG12-AS1 being an enhancer-like, cis regulator of DIRAS3 transcription [51] . The location of these enhancers and their potential specificity for DIRAS3 might explain why GNG12 is not affected by GNG12-AS1 depletion. Another possibility is that GNG12-AS1 expression is limited by GNG12 transcription and its further reduction has no impact on GNG12 expression. An alternative strategy to siRNA for analysing the cis functions of GNG12-AS1 would have been to use CRISPRi, a new technology involving small guide RNAs to recruit a catalytically inactive Cas9 (dCas9) fused to the KRAB transcriptional repressor domain to specific loci [52] . Similar to RNAi, CRISPRi does not affect the underlying gene sequence and was shown to induce transcriptional repression of lncRNAs [52] . However, KRAB-mediated silencing can spread to adjacent genes [53] , which would confound the detection of genes influenced by TI by a lncRNA. Transcription of lncRNA provides an important mechanism for fine-tuning the expression of genes in cis [54] . There is evidence for lncRNAs having a threshold-depended role in moderating gene regulation rather than an activating or repressive role [54] . For example, MALAT1, a lncRNA with several roles in gene regulation, has subtle effects on the expression of its neighbouring genes [55] . A fine-tuning mechanism could explain why small changes in gene expression observed after depletion of some lncRNAs could be relevant upon specific stress or environmental conditions. Imprinted genes are exquisitely regulated for gene dosage. It is likely that in vivo , the cis regulatory function of GNG12-AS1 in fine-tuning DIRAS3 expression is limited to specific developmental stages or environmental conditions as shown for HOTTIP lncRNA [56] , which has similarly low abundance and expression levels. GNG12-AS1 is not imprinted in non-cancer cell lines, as shown previously by pyrosequencing SNP analysis [31] , but our RNA-FISH results indicate that in a substantial proportion of HB2 cells it may be randomly monoallelic. A growing number of autosomal genes are being shown to be randomly monoallelic at single-cell level [57] . If 50% of cells with GNG12-AS1 expression are expressing transcripts from the paternal allele, these would be repressing DIRAS3 in cis by TI, whereas on the other 50% of cells where GNG12-AS1 expression is maternal, DIRAS3 would already be silent on this allele. This would be consistent with the suggestion that random monoallelic expression refines gene expression levels in a population of cells [58] , [59] . In addition to GNG12-AS1 having a cis function in moderating DIRAS3 transcription, GNG12-AS1 also regulates cell cycle progression. Transcriptional upregulation of DIRAS3 induced by GNG12-AS1 depletion led to G1 delay associated with the downregulation of cyclin E1 . As the G1 delay and cyclin E1 levels were rescued by simultaneous depletion of exon 1 siRNA of GNG12-AS1 and DIRAS3 , these data suggest that TI between GNG12-AS1 and DIRAS3 contributes to the regulation of G1 phase of the cell cycle. DIRAS3 was shown to be involved in cell cycle progression [40] , [59] . The upregulation of DIRAS3 by inhibiting GNG12-AS1 transcription in our study does not have the same effect on cyclin genes as previously reported, where DIRAS3 was ectopically overexpressed [40] , [59] , [60] . These differences could be due to the modest upregulation of DIRAS3 induced by transient repression of GNG12-AS1 with siRNA, whereas the latter study ectopically expressed DIRAS3. Nevertheless, our results are consistent with a role for DIRAS3 in cell cycle progression through G1 phase [40] , [59] . More importantly, these results indicate that disruption of TI between GNG12-AS1 and DIRAS3 can have effects on the cell cycle. RNA-FISH analysis indicated that, in addition to co-localization between intronic and exonic probes, we also found cells in which the signals were separated, suggesting that there may be additional functions for GNG12-AS1 . Our cell cycle analysis revealed that GNG12-AS1 depletion with siRNAs to 5′ end and 3′ end resulted in a G2/M delay. This effect is most likely due to a DIRAS3 -independent function of GNG12-AS1 RNA product. This is further supported by our microarray experiments where both siRNAs induced changes in genes involved in cell cycle progression. In addition, we found that reducing the levels of GNG12-AS1 transcripts whether by siRNAs directed to exon 1 or various other exons of GNG12-AS1 resulted in increased cell migration. This phenotype was observed upon GNG12-AS1 knockdown even in cells where DIRAS3 expression was absent. Expression profiling of GNG12-AS1 -depleted cells showed an enrichment for genes involved in cell adhesion, migration and actin cytoskeleton pathways. We were able to validate the upregulation of MET signalling pathway after siRNA-mediated reduction of GNG12-AS1 . MET controls many biological functions such as cell migration, invasion and motility, and its aberrant activation can lead to cancer [41] , [42] , [61] . We have previously shown that GNG12-AS1 is downregulated in breast cancer tumours together with DIRAS3 (ref. 31 ). Thus, it is possible that GNG12-AS1 extends the tumour-suppressor function of this locus by regulating oncogenes such as MET. In keeping with this, MET was recently shown to be regulated by MEG3 lncRNA in pancreatic tumours [62] . Thus, MET could be a common target of lncRNAs involved in the regulation of cellular processes important for tumour growth. Further experiments are necessary to investigate whether the GNG12-AS1 transcript directly interacts with distant genes, and if so whether this interaction is isoform specific. In summary, GNG12-AS1 is similar to several other lncRNAs that have both cis and trans functions [63] , [64] . Although the trans function may be to regulate genes involved in cell cycle and cell migration through direct interaction, the cis function has a role in fine-tuning regulation of DIRAS3 transcription. Altogether, our results demonstrate that an siRNA-based strategy can be employed to successfully separate functions that are due to lncRNA transcription from those of the transcript. Cell culture and treatments HB2 (human mammary epithelial cell line) were cultured in DMEM (GIBCO) supplemented with 10% fetal bovine serum (FBS), 10 ml l −1 penicillin–streptomycin solution, 5 mg ml −1 insulin (Sigma) and 1 mg ml −1 hydrocortisone (Sigma). MCF10A (human breast epithelial cell line) were cultured in MEGM SingleQuots (Lonza). SUM159 (breast cancer cell line) were cultured in Ham’s F-12 medium (GIBCO) supplemented with 5% FBS, 5 mg ml −1 insulin and 1 mg ml −1 hydrocortisone; MCF7 (breast cancer cell line) and HS27 (human foreskin fibroblasts) were cultured in DMEM with 10% FBS and 10 ml l −1 penicillin–streptomycin solution. 293FT cells were grown in DMEM (high glucose 1 × ; GIBCO, ref. 41965039) supplemented with 10% FBS, 0.1 mM MEM Non-Essential Amino Acids (GIBCO), 6 mM L -glutamine (GIBCO), 1 mM MEM Sodium Pyruvate (GIBCO) and 500 μg ml −1 Geneticin (GIBCO). All the cells were from American Type Culture Collection and were cultured at 37 °C with 5% CO 2 . The cells were treated with Actinomycin-D (Sigma) at a final concentration of 10 μg ml −1 for 0, 2, 6, 8 and 24 h. Single-molecule RNA FISH RNA FISH was performed as described [37] . Cells were grown on 18 mm round #1 cover glass, briefly washed with PBS and fixed with PBS/3.7% formaldehyde at room temperature for 10 min. Following fixation, cells were washed two times with PBS. The cells were then permeabilized in 70% ethanol for at least 1 h at 4 °C. Stored cells were briefly rehydrated with Wash Buffer (2 × saline sodium citrate buffer (SSC), 10% formamide) before FISH. The Stellaris FISH Probes ( GNG12-AS1 intronic (Q670) and exonic probes (Q570), sequences in Supplementary Table 1 ) were added to the hybridization buffer (2 × SSC, 10% formamide, 10% dextran sulfate) at the same time to give a final concentration of 250 nM per probe set. Hybridization was carried out in a humidified chamber at 37 °C overnight. The following day, the cells were washed twice with Wash Buffer at 37 °C for 30 min each. The second wash contained 4,6-diamidino-2-phenylindole for nuclear staining (5 ng ml −1 ). The cells were then briefly washed with 2 × SSC and then mounted in Vectashield (Vector Laboratories, H-1000). Images were captured using Nikon TE-2000 inverted microscope with NIS-elements software using a Plan Apochromat × 100 objective and Andor Neo 5.5 sCMOS camera. We acquired 25 optical slices at 0.3 μm intervals. Images were deconvolved with Huygens Professional and projected in two dimensions using Volocity Image Software Analysis. Intronic signals were scored to determine the percentage of cells with mono- or biallelic expression. Exonic signals were then scored on the same cells. To score whether intronic and exonic signals co-localize, we selected cells in which both signals were present. Quantitative real-time PCR RNA (1 μg) was extracted with the RNeasy Kit (QIAGEN) and treated with DNase I (QIAGEN) following the manufacturer’s instructions. QuantiTect Reverse Transcription Kit (QIAGEN) was used for cDNA synthesis including an additional step to eliminate genomic DNA contamination. Quantitative real-time PCR was performed on a 7900HT Fast Real-Time PCR System (Applied Biosystems) with Fast SYBR Green Master Mix (Life Technologies). Thermocycling parameters: 95 °C for 20 s followed by 40 cycles of 95 °C for 1 s and 60 °C for 20 s. Two reference genes ( GAPDH and RPS18 ) were selected. Our microarray data show no significant variation in GAPDH and RPS18 expression in our siRNA experiments in HB2, HS27 and SUM159 cells. Expression levels of GNG12-AS1 , DIRAS3, GNG12 and WLS in non-cancer and cancer cell lines are normalized relative to the geometric mean of GAPDH and RPS18 ( Supplementary Fig. 1a ). The expression levels using either GAPDH ( Fig. 2c,d and Supplementary Fig. 3a,b ) or the average of GAPDH and RPS18 ( Supplementary Fig. 3c–f ) across siRNA conditions were consistent and reproducible. Thus, we used only GAPDH normalization for further experiments. Exon 7–8 of GNG12-AS1 was used to quantify its expression, if not stated otherwise. To calculate the GNG12-AS1 copy number, standard curve of Ct values was performed by qRT–PCR using dilution series of known concentration of GNG12-AS1 DNA template (variant 1 that contains exon 1, 2, 3, 4, 5, 6, 7, 8, 8b and 9). cDNA was made from RNA extracted from known number of different cell lines. The Ct values were fitted on the standard curve and the number of GNG12-AS1 molecules per cell was calculated. The final value was multiplied by 2, to account for the fact that cDNA is single stranded and DNA templates used to make standard curve is double stranded. The sequences for expression primers are listed in Supplementary Table 2 . The amplification efficiency of housekeeping genes was measured with serial dilution of cDNA of each gene from five different cell lines. PCR efficiencies and correlation coefficients (R2) for each primer pair are shown in Supplementary Table 3 . RNA interference The sequences of siRNAs are present in the Supplementary Table 4 . The cells were transfected with DharmaFECT 1 (SUM159, MCF7, MCF10A), DharmaFECT 3 (HS27) or DharmaFECT 4 (HB2) (Thermo-Scientific) following the manufacturer’s instructions. All experiments were done 48 h after transfection and all the siRNAs were used at a final concentration of 50 nM. siRNA-mediated depletion of GNG12-AS1 RNA and proteins were fractionated as described previously [65] . The cells were either untreated (for immunoblot analysis) or transfected with control and GNG12-AS1 siRNAs (for RNA analysis). RNA was isolated from cytoplasmic, nucleoplasmic and chromatin fractions by TRIZOL extraction (Life Technologies) and used for qRT–PCR. Data were normalized to the geometric mean of GAPDH and β-actin levels in each cellular compartment as no normalization controls is equal in all three compartments (for details see ref. 65 ). MALAT1 and RPS18 were used as positive controls for chromatin and cytoplasmic fractions, respectively. Primers used for this assay are listed in Supplementary Table 2 . Nuclear run-on assay Nuclear run-on assay was performed as described previously [66] . Cells were grown in 10 cm dishes, trypsinized and centrifuged, and the pellets were washed with 1.5 ml of NP-40 lysis buffer (10 mM Tris-HCl, 10 mM NaCl, 3 mM MgCl 2 , 0.5% NP-40), incubated on ice for 5 min and centrifuged at 1,500 g for 5 min. Pellets were then washed again with 1.5 ml NP-40 lysis buffer. The nuclei pellets were resuspended in 70 μl glycerol storage buffer (50 mM Tris-HCl, pH 8, 0.1 mM EDTA, 5 mM MgCl 2 , 40% glycerol) and flash frozen in liquid nitrogen. 60 μl were transferred to fresh nuclease-free tubes and equal amount of the 2 × run-on transcription buffer (20 mM Tris-HCl, pH8; 5 mM MgCl 2 , 300 mM KCl, 4 mM dithiothreitol) was added together with 2 mM ATP, CTP, GTP (GE Healthcare) and 1 mM Biotin-16-UTP (Epicentre). The reaction was incubated at 30 °C for 45 min. In vitro transcription was stopped by adding TURBO DNase (Ambion) at 37 °C for 30 min. Then 100 μl of nuclei lysis buffer (50 mM Tris-HCl, pH 7.5; 5% SDS, 0.125 M EDTA) and Proteinase K (Ambion) were added to the sample and incubated at 37 °C for 30 min. RNA extraction was performed using phenol/chloroform/isoamyl alcohol: 25:24:1 (Invitrogen) and chloroform/isoamyl alcohol: 24:1 (Sigma). To precipitate RNA, 3 M sodium acetate pH 5.5 (Life Technologies), GlycoBlue (Life Technologies) and ice-cold 100% ethanol were added. The samples were incubated at −80 °C for 30 min and centrifuged at 12,000 g for 15 min. Pellets were washed with ice-cold 70% ethanol and centrifuged at 12,000 g for 10 min. The pellets were then resuspended in 30 μl nuclease-free water. RNA samples were then purified on column using RNeasy kit (Qiagen) to remove free Biotin-16-UTPs, according to the manufacturer’s instructions. Purified RNA from column was eluted in 30 μl nuclease-free water. Biotinylated RNA from samples was captured using Dynabeads MyOne C1 streptavidin beads (Invitrogen). C1 beads (40 μl per sample) were washed twice with Solution A (100 mM NaOH, 50 mM NaCl) for 3 min and once with Solution B (100 mM NaCl). The C1 beads were then preblocked with BSA (200 μg ml −1 ) and Yeast tRNA (200 μg ml −1 ; Invitrogen) mix in Solution B. The beads were pre-blocked on a rotor at room temperature for 30 min, collected on magnetic stand and resuspended in Solution B. Beads were aliquoted into nuclease-free tubes and equal amount (20 μl) of RNA was added. Biotinylated RNA was pulled down for 2 h at room temperature. Then the beads were collected on magnetic stand, washed three times with 1 × Wash/Binding buffer (2 × Wash/Binding buffer: 10 mM Tris-HCl, pH 7.4; 1 mM EDTA, 2 M NaCl). After the final wash, C1 beads with bound RNA were eluted in 30 μl nuclease-free water and used directly for reverse transcription to prepare cDNA. Relative transcription was calculated as: 2^ −[MeanCt(gene)-MeanCt(β-actin)]. For GNG12-AS1 knockdown experiments, control transcription was set to 1. β-Actin primer was used for normalization (primers are listed in Supplementary Table 2 ). Lentivirus overexpression of GNG12-AS1 in human cells The different GNG12-AS1 splice variants and negative control vector (scrambled sequence) were first cloned in pJET1.2 plasmid (Fermentas) and then into modified pLenti6.3/TO/V5-DEST vector (kindly provided by John Rinn, Harvard University) using Gateway cloning strategy. The sequences are listed in Supplementary Data 1 . The modified vector does not contain WPRE, the SV40 promoter and the blasticidin-resistance gene that could interfere with lncRNA structure and function. Sanger sequencing and restriction digestion using PvuI-HF and BsrGI enzymes confirmed the GNG12-AS1 inserts. Lentiviral transduction of GNG12-AS1 clones was done in 293FT cells using ViraPower (Invitrogen) including, negative and positive control vector containing mCherry. The DNA-Lipofectamine2000 complexes were added to 293FT cells and incubated overnight. Forty-eight and seventy-two hours post transfection, the virus-containing supernatants were harvested, centrifuged at 700 g for 5 min at 4 °C and filtered with 0.45 μm with additional 0.22 μm filter before being stored at 4 °C. To transduce SUM159 cells, 80,000 cells per 12-well plate were seeded in triplicate and transduced with the lentiviruses at a multiplicity of infection of 0.1 together with polybrene (5 μg ml −1 , Sigma). Transduction efficiency (>80%) was verified using positive control vector containing mCherry and measured by FACS Calibur Influx (Beckton Dickinson) using BDFACS Software 1.0.0.650. The FACS data were analysed using FlowJo software (TreeStar Inc). Exon 7–9 of GNG12-AS1 was used to quantify its overexpression (primers are listed in Supplementary Table 2 ). Microarray analysis Gene expression analysis was carried out on Illumina Human HT12 version 4 arrays. All data analyses were carried out on R using Bioconductor packages [67] . Raw intensity data from the array scanner were processed using the BASH [68] and HULK algorithms as implemented in the bead array package [69] . Log2 transformation and quantile normalization of the data were performed across all sample groups. Differential expression analysis was carried out using the Limma package [70] . Differentially expressed genes were selected using a P -value cutoff of <0.05 after application of FDR correction for multiple testing applied globally to correct for multiple contrasts. RNA was extracted from cells (HB2, SUM159) treated with control and GNG12-AS1 siRNAs (exons 1 and 7). The analysis was performed with six biological replicates for each cell line. cDNA synthesis, labelling and array procedure were conducted at the Genomic Facility at the CRUK CI. Pathway analysis was performed using Metacore. MeDIP (methylated DNA immunoprecipitation) qRT–PCR Genomic DNA was extracted from cells with control and GNG12-AS1 siRNA treated with 100 μg ml −1 RNaseA (Invitrogen) in 100 μl of Tris-EDTA for 10 min at room temperature and sonicated for 5 min (Diagenode Picoruptor, 30 s ON-30sec OFF) to obtain an average fragments size of 300 bp. DNA was purified using 1.8 volumes AMPURE XP beads (Beckman Coulter) according to the manufacturer’s instructions and resuspended in 185 μl of water. The samples were boiled for 10 min and snap frozen on ice for 10 min. Five microlitres were taken as input followed by addition of 20 μl cold 10 × meDIP buffer. Meanwhile, 20 μl of Protein G Dynal beads (Invitrogen) were blocked with PBS/0.01% BSA for 30 min at room temperature and washed three times with 1 × meDIP buffer. One microlitre of anti-5mC antibody (Diagenode) was conjugated to the washed beads in 200 μl of 1 × meDIP buffer for 2 h at room temperature. Antibody-bead conjugates were washed three times with cold 1 × meDIP buffer, added to the sample DNA and incubated overnight at 4 °C in an overhead rotator. The bound material was washed three times with 200 μl of 1 × meDIP buffer at room temperature. Bound and input material were resuspended in 50 μl lysis solution (100 mM Tris-HCl, pH 5.5, 5 mM EDTA, 200 mM NaCl, 0.2% SDS plus 20 μg proteinase K (Invitrogen 25530-049)) and incubated at 60 °C for 30 min. DNA was purified using 1.8 volumes AMPURE XP beads (Beckman Coulter) according to the manufacturer’s instructions. Validation of Medip was done by qRT – PCR. The list of Medip primers is present in Supplementary Table 2 . Analysis of allelic expression and DNA methylation Analysis of DNA methylation was by bisulfite conversion with the EZ DNA Methylation-Gold Kit (Zymo Research) and subsequent pyrosequencing as described [31] . The list of primers used for this experiment is present in Supplementary Table 5 . RNA immunoprecipitation HB2 cells were transfected with control and GNG12-AS1 siRNAs and RIP was performed from nuclear extracts using mouse IgG (Cell Signaling) and AGO2 (Abcam) antibodies. Quality of cytoplasmic and nuclear extracts was assessed by immunoblot as described previously [65] . Eight micrograms of antibody were incubated with 70 μl of Dynabeads Protein G beads (Life Technologies) in total volume of 280 μl for 30 min at room temperature. The antibody–bead complex was incubated with 500 μg of nuclear exactas for 2–3 h at 4 °C and then washed three times (5 min each) with equal amount of 1 × NLB buffer (20 mM Tris-HCl, pH7.5, 0.15 M NaCl, 3 mM MgCl 2 , 0.3% NP-40, 10% glycerol) supplemented with Complete EDTA free protease inhibitor cocktail (14549800; Roche) and phosphatase inhibitors (1 mM NaF, 1 mM Na 3 VO 4 ) and RNAse OUT (100 U; Life Technologies). The RNA was extracted by addition of 1 ml TRIzol (Life Technologies) to the beads, followed by 1/5 volume of Chloroform (Sigma). 10% of the input lysate was mixed with 1 ml of TRIzol for the total input RNA. After centrifugation at 12,000 g for 15 min at 4 °C, the aqueous supernatant was transferred to a new tube and RNA was precipitated with 1/10 volume of 3 M sodium acetate pH 5.5 (Life Technologies), 1 volume of isopropanol (Sigma) and 1 μl of GlycoBLue (Life Technologies) at −80 °C for 20 min. After 30 min centrifugation at 12,000 g at 4 °C, the RNA pellet was washed twice with ice-cold 70% ethanol. Finally, the pellet was dissolved in 15 μl of RNAse-free water (Life Technologies). We used Power SYBR Green RNA-to-CT 1-Step Kit (Life Technologies) for qRT–PCR. Primers for this assay were GNG12-AS1 (exons 7–8) and U1 and GAPDH (negative controls for AGO2 binding). Primers are listed in Supplementary Table 2 . Cell lysis and immunoblot Total cell lysis and immunoblot were performed as described previously [31] . Briefly, the cells were lysed in lysis buffer (50 mM Tris-HCl, pH 8, 125 mM NaCl, 1% NP-40, 2 mM EDTA, 1 mM phenylmethylsulphonyl fluoride, and protease inhibitor cocktail (Roche)) and incubated on ice for 25 min. The proteins were denatured, reduced and separated using Nupage Novex 4–12% Bis-Tris Protein Gels (Invitrogen). Secondary antibodies were conjugated with peroxidase, and immunobands were detected with a Supersignal West Dura HRP Detection Kit (Thermo-Scientific). Quantification of immunoblots was done on ImageScanner III (GE HealthCare) using the software package ImageQuant TL 7.0 (GE HealthCare). Uncropped scans of the immunoblots are shown in Supplementary Fig. 12 . Antibodies The list of antibodies is present in Supplementary Table 6 . Chromatin immunoprecipitation ChIP assays were performed as previously described [31] with antibodies listed in the Supplementary Table 6 . The input and the immunoprecipitated materials were quantified by QubitFluorometer (Life Technologies) with the dsDNA BR Assay Kit (Invitrogen). Thirty micrograms of chromatin and 5 μg of antibody were used for ChIP experiment. The qPCR data were corrected for DNA amount, and enrichment was normalized against the input according to the formula 2-dCt(Ab)—log2(DF)]—[Ct(input)—log2(DF)]. Primer sequences are present in Supplementary Table 2 . Cell synchronization The HB2 cells were plated in six-well plates and 24 h later thymidine (2 mM) was added. The cells were incubated for 18 h, washed three times with PBS and released into thymidine-free medium for 9 h. Thymidine was then added for a further 15 h. The cells were then washed three times with PBS. At this point, the cells in G1/S phase were collected for RNA, FACS and protein analysis (T0) in a serum-rich medium without thymidine. Time points were collected 3 (T3), 8 (T8), 14 (T14), 24 (T24) and 32 (T32) hours later. In the case of serum starvation, HB2 cells were plated in six-well plates and then switched to serum-free medium for 48 h. After starvation (T0), the cells were released into cell cycle by addition of serum and the time points for RNA and protein analysis were collected at 3 (T3), 6 (T6), 10 (T10), 15 (T15) and 34 (T34) hours. Cyclin E1 (G1/S transition marker) levels were used to monitor cell cycle progression by immunoblot. In the case of siRNA treatment, the cells were first transfected with siRNAs and thymidine was added 24 h later for additional 18 h. The procedure was continued as described above. Cell cycle analysis The HB2 cells were transfected with siRNAs and harvested after 72 h, washed with PBS and fixed with 70% ethanol (the samples were stored for up to 1 week at 4 °C). The cells were then washed once with PBS, incubated in PBS containing RNase A (100 μg ml −1 , Life Tecnologies) for 30 min at 37 °C, stained with propidium iodide (20 μg ml −1 , Life Tecnologies) and incubated on ice in the dark for 30 min. DNA content was analysed by FACS Calibur (Beckton Dickinson) using BD CellQuest Pro Software V6. DNA cell cycle analysis was performed on FlowJo software V9 (TreeStar Inc) to quantify cell cycle distribution. Wound healing assay Wound healing assay was performed on 24-well (Essen Imagelock) plates in triplicates after treatment of cells with control and siRNAs against GNG12-AS1 . Forty-eight hours after siRNA treatment, scratch wounds were induced with 10 μl sterile pipette tip, after which fresh culture medium was added. The IncuCyte 2011A Rev2 software was used to capture and analyse the pictures. The cell migration was followed in time for 24 h using IncuCyte FLR (Essen Bioscience), making measurements in triplicate every 3 h. Statistical analysis The statistical significance of data was determined by two-tailed Student’s t -test in all experiments using GraphPad Prism unless indicated otherwise. P -values>0.05 were considered statistically not significant. Accession codes: The microarray data have been deposited in the Gene Expression Omnibus of National Center for Biotechnology Information under the accession number GSE60563 . How to cite this article: Stojic, L. et al. Transcriptional silencing of long noncoding RNA GNG12-AS1 uncouples its transcriptional and product-related functions. Nat. Commun. 7:10406 doi: 10.1038/ncomms10406 (2016).